Syntenin-ALIX exosome biogenesis and budding into multivesicular bodies are controlled by ARF6 and PLD2 Exosomes are small vesicles that are secreted by cells and act as mediators of cell to cell communication. Because of their potential therapeutic significance, important efforts are being made towards characterizing exosomal contents. However, little is known about the mechanisms that govern exosome biogenesis. We have recently shown that the exosomal protein syntenin supports exosome production. Here we identify the small GTPase ADP ribosylation factor 6 (ARF6) and its effector phospholipase D2 (PLD2) as regulators of syntenin exosomes. ARF6 and PLD2 affect exosomes by controlling the budding of intraluminal vesicles (ILVs) into multivesicular bodies (MVBs). ARF6 also controls epidermal growth factor receptor degradation, suggesting a role in degradative MVBs. Yet ARF6 does not affect HIV-1 budding, excluding general effects on Endosomal Sorting Complexes Required for Transport. Our study highlights a novel pathway controlling ILV budding and exosome biogenesis and identifies an unexpected role for ARF6 in late endosomal trafficking. After internalization, cell surface molecules can follow different trafficking routes. For example, from early endosomes they can be sorted for recycling to the plasma membrane or degradation in lysosomes. The formation and the maturation of endosomes are essential in regulating this traffic. During maturation, inward invagination of the limiting membrane of the endosome gives rise to intraluminal vesicles (ILVs). The late endosome is then called a multivesicular body or MVB [1] . This vesiculation has been shown to increase upon signalling via growth factor receptors, and the inclusion in ILVs inactivates signalling receptors because it deprives them from contact with the cytosol [2] . MVBs move towards the perinuclear area of the cell where they can directly fuse with lysosomes creating hybrid organelles, where endocytosed cargos are degraded [3] . Alternatively, MVBs can fuse with the plasma membrane inducing the secretion in the extracellular environment of ILVs that will be now called exosomes. Exosomes are proposed to function as mediators of intercellular communication and might lead to reprogramming of recipient cells [4] , [5] . Multiple pathways seem to operate on endosomal membranes and give rise to different populations of MVBs. Different populations of ILVs, enriched in different lipids, can coexist [6] and form within single MVBs that can be distinguished on the basis of size and mechanism of formation [7] . The mechanisms of ILV formation and sorting of endosomal proteins into these vesicles are partially understood. The best described machinery that drives ILV formation into MVB is the endosomal sorting complexes required for transport (ESCRT) machinery. In this pathway, ILV formation requires ubiquitination and the sequential action of different components of the ESCRT [8] , [9] , [10] . Yet ubiquitin and ESCRT-independent pathways have also been identified and might coexist with ESCRT-dependent machinery attesting for different MVB subpopulations fated for either lysosomal degradation or exosomal release [11] , [12] , [13] . A population of exosomes requires neutral sphingomyelinase 2 to produce ceramide, thereby forming raft-based microdomains [14] . Higher-order oligomerization of membrane complexes might also drive exosome formation [15] . We have recently shown that the PDZ protein syntenin stimulates exosome production and is required for the budding of CD63-positive ILVs into MVBs [16] . Syntenin is highly enriched in exosomes (ExoCarta exosome database www.exocarta.org ), and the stimulation of exosome production by syntenin depends on the interaction of its N-terminal domain with ALIX [16] , an auxiliary component of the ESCRT machinery that supports viral budding [17] , [18] . Syntenin interaction with ALIX mimics retroviral late domain protein–ALIX interaction [16] , which is known to be essential for efficient retroviral budding [18] . The production of syntenin exosomes requires certain ESCRTs components (that is, VPS22 and CHMP2A) but is independent of others (CHMP3 and CHMP6) [16] . This suggests that the biogenesis of exosomes might use alternative ESCRT pathways. Importantly, syntenin PDZ domains directly bind to multiple membrane receptors such as syndecans [19] and the tetraspanin CD63 (ref. 20 ), supporting their exosomal sorting [16] . We have previously found that syntenin interacts genetically with the small GTPase ADP-Ribosylation Factor 6 (ARF6), and that syntenin-ARF6 interaction is crucial for early polarized movements during zebrafish development [21] . ARF6 is localized at the plasma membrane and on endosomes, and regulates membrane transport, vesicular trafficking (endocytosis, recycling and exocytosis) and membrane remodelling by regulating actin cytoskeleton and phosphoinositides metabolism [22] , [23] . Like other small GTPases, ARF6 works as a molecular switch that cycles between the active (GTP-bound) and inactive (GDP-bound) state, and ARF6 function is under tight spatial control, which is mediated by guanine nucleotide exchange factors (GEFs) that catalyse GTP exchange [23] . Activated ARF6 has been shown to function through activation of two major effectors, Phosphatidylinositol 4-Phosphate 5-Kinase (PIP5K) and Phospholipase D (PLD) [24] , [25] . We have shown that ARF6 and its effector PIP5K control the endocytic recycling of syntenin PDZ-interactors, that is, syndecans, in a phosphatidylinositol 4,5-bisphosphate-dependent manner and that this pathway is important for cell spreading [26] . Here, testing for the impact of ARF6 on syntenin exosomes, we identify ARF6 as a regulator of ILV budding and exosome production. We show that these effects rely on the ARF6 effector PLD2. These findings depict a role for ARF6 in late endosomal events and contribute to our understanding of the mechanisms of exosome biogenesis at the level of ILV budding. ARF6 regulates exosomes Because of the genetic interaction between ARF6 and syntenin and because ARF6-syntenin is involved in endosomal trafficking, we investigated the role of ARF6 on the production of syntenin exosomes. We used MCF-7 cells as a model, in which ‘syntenin-exosomes’ represent up to 50% of the secreted particles [16] . Moreover, MCF-7 cell secreted particles pelleted by high-speed centrifugation (HSC) are exosomal-like in size (~88 nm diameter), and syntenin and associated proteins (Syndecans, CD63, ALIX) are exclusively present in the exosomal fraction as determined by density gradient experiments [16] . Two different RNA-mediated interference (RNAi) molecules were used to efficiently knock down ARF6, as compared with cells incubated in the presence of a control (CNT) RNAi ( Fig. 1a ). ARF6 depletion did not have an impact on cell growth or density and did not significantly affect the levels of syntenin, ALIX or syndecan-1 C-terminal fragment (SDC1CTF) but nearly doubled the amount of CD63 in cells ( Fig. 1a,b ). Exosomes were isolated from control and ARF6-depleted cells by HSC and were analysed by western blot ( Fig. 1c,d ). The two different RNAis targeting ARF6 induced a significant decrease in several exosomal proteins, such as syntenin (down to 27 and 22% of the control levels), ALIX (27 and 46% of the control levels), CD63 (54 and 60% of the control levels) and SDC1CTF (30 and 22% of the control levels) ( Fig. 1d ), suggesting that ARF6 expression is required for exosome production. 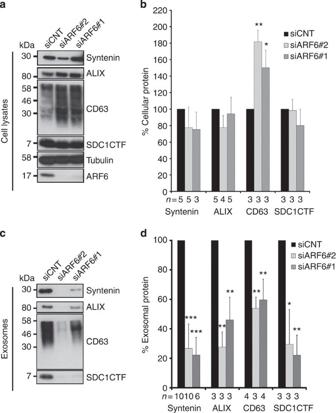Figure 1: ARF6 depletion decreases syntenin exosome release. MCF-7 cells were treated with 2 different ARF6 RNAi (siARF6#1 and siARF6#2) or non-targeting RNAi (siCNT). Total cell lysates (a) and the corresponding exosomes (c) were analysed by western blotting for different markers, as indicated. Histograms represent mean signal intensities±s.d. in cell lysates or exosomes, relative to signals in siCNT cells or exosomes, calculated fornindependent experiments (b,d). SDC1CTF; syndecan-1 C-terminal fragment. *P<0.05, **P<0.01, ***P<0.001 (Student’st-test). Figure 1: ARF6 depletion decreases syntenin exosome release. MCF-7 cells were treated with 2 different ARF6 RNAi (siARF6#1 and siARF6#2) or non-targeting RNAi (siCNT). Total cell lysates ( a ) and the corresponding exosomes ( c ) were analysed by western blotting for different markers, as indicated. Histograms represent mean signal intensities±s.d. in cell lysates or exosomes, relative to signals in siCNT cells or exosomes, calculated for n independent experiments ( b , d ). SDC1CTF; syndecan-1 C-terminal fragment. * P <0.05, ** P <0.01, *** P <0.001 (Student’s t -test). Full size image To complement these loss-of-function studies, we overexpressed the wild-type form of ARF6 (ARF6-WT) and a fast-cycling mutant (ARF6-T157N) ( Fig. 2a ). ARF6 overexpression did not affect the expression of syntenin, ALIX or CD63 in the cell lysates ( Fig. 2a ). Exosomes (HSC pellet) from control and overexpressing cells were analysed by western blot ( Fig. 2b ). The overexpression of the fast-cycling mutant ARF6-T157N significantly enhanced exosomal release of syntenin (195%), ALIX (167%) and CD63 (131%), whereas overexpression of ARF6-WT had no significant effect ( Fig. 2a,b ). Finally, the effects of ARF6 silencing were partially prevented by overexpression of ARF6-T157N ( Supplementary Fig. 1a,b ). Taken together, these data reveal the importance of ARF6 and its GDP/GTP cycling for syntenin exosomal production. 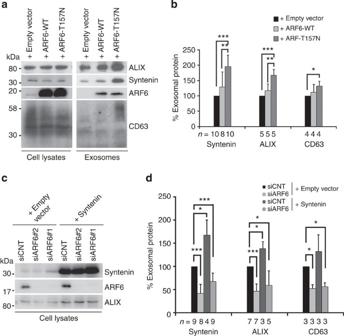Figure 2: ARF6 and ARF6 cycling are required for syntenin exosome release. MCF-7 cells were transiently transfected with an expression vector for wild-type ARF6 (+ARF6-WT), an expression vector for the fast cycling mutant of ARF6 (+ARF6-T157N) or the empty vector (pCDNA3) as control. (a) Total cell lysates and corresponding exosomes were collected 24 h after transfection and analysed by western blotting for different markers, as indicated. (b) Histograms represent mean±s.d. signal intensities in exosomes, relative to signals in siCNT exosomes, calculated fornindependent experiments. (c) MCF-7 cells were treated with ARF6 RNAi (siARF6#2 and siARF6#1) or non-targeting RNAi (siCNT) for 48 h and then transiently transfected with an expression vector for wild-type syntenin (+ Syntenin) or the empty vector (pCDNA3) as control. Total cell lysates (c) and corresponding exosomes (d) were collected 24 h after transfection and analysed by western blotting for different markers, as indicated. (d) Histograms represent mean signal intensities±s.d. in exosomes, relative to signals in siCNT exosomes, calculated fornindependent experiments. siARF6#1 and siARF6#2 data were pooled for quantification and statistical analysis. *P<0.05, **P<0.01, ***P<0.001 (Student’st-test). Figure 2: ARF6 and ARF6 cycling are required for syntenin exosome release. MCF-7 cells were transiently transfected with an expression vector for wild-type ARF6 (+ARF6-WT), an expression vector for the fast cycling mutant of ARF6 (+ARF6-T157N) or the empty vector (pCDNA3) as control. ( a ) Total cell lysates and corresponding exosomes were collected 24 h after transfection and analysed by western blotting for different markers, as indicated. ( b ) Histograms represent mean±s.d. signal intensities in exosomes, relative to signals in siCNT exosomes, calculated for n independent experiments. ( c ) MCF-7 cells were treated with ARF6 RNAi (siARF6#2 and siARF6#1) or non-targeting RNAi (siCNT) for 48 h and then transiently transfected with an expression vector for wild-type syntenin (+ Syntenin) or the empty vector (pCDNA3) as control. Total cell lysates ( c ) and corresponding exosomes ( d ) were collected 24 h after transfection and analysed by western blotting for different markers, as indicated. ( d ) Histograms represent mean signal intensities±s.d. in exosomes, relative to signals in siCNT exosomes, calculated for n independent experiments. siARF6#1 and siARF6#2 data were pooled for quantification and statistical analysis. * P <0.05, ** P <0.01, *** P <0.001 (Student’s t -test). Full size image In an attempt to clarify whether specific ARF6 GEFs are implicated in syntenin exosome production, the roles of ARNO, GEP100 and EFA6, three GEFs expressed in MCF-7 cells were investigated ( Supplementary Fig. 2a ). EFA6D is the most highly expressed isoform of EFA6 in MCF-7 cells, consistent with previous results showing the widespread tissue distribution of EFA6D compared with the other isoforms [27] . Efficient silencing of ARNO, GEP100 and EFA6D expression (75, 85 and 93% depletion, respectively, Supplementary Fig. 2b ) decreased syntenin exosome production ( Supplementary Fig. 2c–e ). Yet, GEP100 and EFA6D silencing also decreased syntenin levels in the cell lysates making the interpretation of the results for these two GEFs difficult. In overexpression experiments, only ARNO induced a significant increase in syntenin exosomal secretion ( Supplementary Fig. 2f–h ), suggesting that ARNO is involved in exosome production. We previously described that MCF-7 cells overexpressing syntenin secrete more exosomes and exosomal markers such as syntenin or CD63 (ref. 16 ). Interestingly, the depletion of ARF6 in cells largely prevents exosome stimulation induced by syntenin overexpression ( Fig. 2c,d ). These results also indicate that ARF6 function is essential for syntenin exosome production. ARF6 is implicated in ILV budding As ARF6 is involved in endocytosis [22] , [23] , we wondered whether ARF6 silencing was precluding components from reaching the endosomal compartment. We therefore investigated the internalization of CD63, a syntenin PDZ ligand and a bona fide exosomal marker, by an antibody uptake from the plasma membrane. We observed no increase in CD63 signal at the plasma membrane of ARF6-depleted cells, and kinetic experiments revealed that ARF6 depletion did not significantly affect CD63 internalization ( Fig. 3a and Supplementary Fig. 3a,b ). 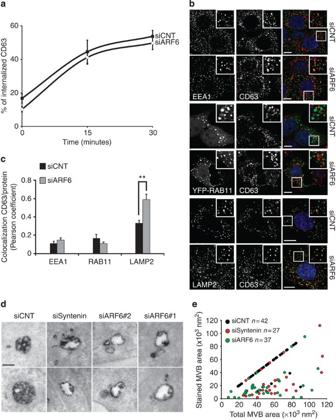Figure 3: ARF6 regulates CD63 late endosomal trafficking. (a) MCF-7 cells were treated with ARF6#1 RNAi (siARF6) or non-targeting RNAi (siCNT). The internalization of the CD63 antibody was monitored by confocal microscopy analysis after 0, 15 and 30 min. The fraction of total CD63 internalized was measured using 10 to 20 cells, taken from two independent experiments (seeSupplementary Fig. 3a,bfor illustrations). The graph illustrates the mean percentage of intracellular CD63 signal, the bars correspond to s.d. (b) Representative confocal micrographs showing the steady-state subcellular distribution of endogenous CD63 together with that of endogenous EEA1, overexpressed eYFP-RAB11 or endogenous LAMP2, in CNT cells and in ARF6-depleted cells (ARF6#2 RNAi). See insets for high magnification ( × 3). Note the high level of co-localization of CD63 with LAMP2, not with EEA1 or eYFP-RAB11 in ARF6-depleted cells. In the merge, CD63 is in red, nuclei were stained with Hoechst (blue), and endosomal markers are in green. Scale bar, 10 μm. (c) CD63 colocalization with EEA1, RAB11 and LAMP2 was assessed by calculating the Pearson correlation coefficient on 10 cells per condition using the JACoP plugin on ImageJ. Histograms represent the mean Pearson coefficient±s.d. in ARF6-depleted cells, relative to signals in siCNT cells, calculated for three independent experiments. **P<0.01 (Student’st-test). (d) Representative electron micrographs, illustrating the morphology of the late endosomal compartment in MCF-7 cells treated with control, syntenin or 2 different ARF6 RNAi, as indicated. Structures were revealed by peroxidase-conjugated anti-CD63 internalized for 30 min, and staining with DAB. Scale bar, 200 nm. (e) Endosome filling. For each peroxidase/DAB-marked endosome, the stained sectional area of the endosome is plotted against the total sectional area of that endosome. siARF6#1 and siARF6#2 data were pooled,nis the total number of endosomes examined in four independent experiments. Figure 3: ARF6 regulates CD63 late endosomal trafficking. ( a ) MCF-7 cells were treated with ARF6#1 RNAi (siARF6) or non-targeting RNAi (siCNT). The internalization of the CD63 antibody was monitored by confocal microscopy analysis after 0, 15 and 30 min. The fraction of total CD63 internalized was measured using 10 to 20 cells, taken from two independent experiments (see Supplementary Fig. 3a,b for illustrations). The graph illustrates the mean percentage of intracellular CD63 signal, the bars correspond to s.d. ( b ) Representative confocal micrographs showing the steady-state subcellular distribution of endogenous CD63 together with that of endogenous EEA1, overexpressed eYFP-RAB11 or endogenous LAMP2, in CNT cells and in ARF6-depleted cells (ARF6#2 RNAi). See insets for high magnification ( × 3). Note the high level of co-localization of CD63 with LAMP2, not with EEA1 or eYFP-RAB11 in ARF6-depleted cells. In the merge, CD63 is in red, nuclei were stained with Hoechst (blue), and endosomal markers are in green. Scale bar, 10 μm. ( c ) CD63 colocalization with EEA1, RAB11 and LAMP2 was assessed by calculating the Pearson correlation coefficient on 10 cells per condition using the JACoP plugin on ImageJ. Histograms represent the mean Pearson coefficient±s.d. in ARF6-depleted cells, relative to signals in siCNT cells, calculated for three independent experiments. ** P <0.01 (Student’s t -test). ( d ) Representative electron micrographs, illustrating the morphology of the late endosomal compartment in MCF-7 cells treated with control, syntenin or 2 different ARF6 RNAi, as indicated. Structures were revealed by peroxidase-conjugated anti-CD63 internalized for 30 min, and staining with DAB. Scale bar, 200 nm. ( e ) Endosome filling. For each peroxidase/DAB-marked endosome, the stained sectional area of the endosome is plotted against the total sectional area of that endosome. siARF6#1 and siARF6#2 data were pooled, n is the total number of endosomes examined in four independent experiments. Full size image We then investigated the localization of CD63 in ARF6-depleted cells by confocal microscopy, together with that of various markers of the endocytic pathway. CD63 staining presented a punctate distribution that partially colocalized with the early endosomal marker EEA1 and the recycling marker RAB11, in either control or ARF6-depleted cells. CD63 also partially colocalized with the lysosomal marker LAMP2 (lysosomal-associated membrane protein) in control cells, but this colocalization was significantly enhanced in ARF6-depleted cells ( Fig. 3b,c ). These data suggest that ARF6 depletion did not block the trafficking of CD63 in early or recycling endosomes, but blocks CD63 in late endosomal compartments. The localization of endogenous ARF6 on late endosomes and MVBs could not be investigated because of the lack of anti-ARF6 antibodies for microscopy experiments. As an approximation, we looked at the localization of fluorescently tagged ARF6. We used the overexpression of RAB5(Q79L), which impairs endosomal trafficking, and induced the formation of enlarged endosomes with a large number of ILVs inside [28] . Overexpressed ARF6 decorates the limiting membrane of RAB5(Q79L)-enlarged endosomes ( Supplementary Fig. 3c ). This suggests a role for ARF6 at the limiting membrane of MVBs. We also investigated the role of the different GEFs in endosomal budding into RAB5(Q79L)-enlarged endosomes. Proteins that normally bud inside MVBs are expected to be found inside these enlarged RAB5(Q79L) endosomes. Consistently, mCherry-syntenin (mCh-syntenin) accumulates inside the lumen of Cerulean-RAB5(Q79L) (Ce-RAB5(Q79L))-decorated enlarged endosomes [16] . Confocal microscopy revealed that mCh-syntenin fills the lumen of many Ce-RAB5(Q79L) endosomes in MCF-7 cells depleted for GEP100 or EFA6D (84% and 74% respectively Supplementary Fig. 3d,e ), suggesting that these ARF6 activators are not involved in the ILV budding in the ARF6-syntenin-exosomal pathway. In contrast, ARNO depletion drastically reduced mCh-syntenin enrichment inside Ce-RAB5(Q79L) endosomes, yielding only 50% mCh-syntenin filled endosomes ( Supplementary Fig. 3d,e ). These results point again to a potential role for ARNO in the ARF6 exosomal pathway. To investigate the role of ARF6 in late endosomal trafficking, we performed electron microscopy experiments looking at the trafficking of CD63 to MVB. We monitored the localization of anti-CD63:HRP conjugates using peroxidase cytochemistry after 30 min internalization. The size of the stained vesicles was not affected, but MVB morphology was clearly altered in ARF6-depleted cells. In control cells, diaminobenzidine (DAB) staining was found on limiting endosomal membranes and in close association with ILVs, filling up the lumen of endosomes ( Fig. 3d , left images). In contrast, in ARF6-depleted cells, the staining was associated with limiting membranes and with ILVs that were peripherally located, the lumen of the endosomes remaining largely empty ( Fig. 3d,e ). This was reminiscent of the MVB morphology in syntenin RNAi-treated cells [16] ( Fig. 3d,e ). These electron microscopy experiments indicate that ARF6 has an impact on ILV budding in endosomes to form MVB and support a role for ARF6 in exosome biogenesis. ARF6 controls EGFR degradation Despite the large literature on ARF6, to our knowledge, this small GTPase has never been implicated in late endosomal sorting [29] . To clarify the functional specificity of ARF6 in late endosomal trafficking, we tested whether ARF6 might also influence sorting and/or degradation of MVB cargo destined for lysosomal degradation. Receptor protein targeting for degradation through the MVB pathway classically depends on ligand-stimulation, ubiquitination and ESCRTs [10] . EGFR sorting to ILVs/MVBs before its lysosomal degradation upon EGF stimulation is the paradigm of such ESCRT-dependent pathway. Interestingly, in ARF6-depleted cells, the degradation of EGFR induced by EGF stimulation was strongly reduced compared with controls ( Fig. 4a,b ). Consistently, the cellular level of EGFR was significantly higher in ARF6-depleted cells ( Fig. 4c ). EGFR was not released in exosomes ( Supplementary Fig. 4a ), indicating that the increased amount of EGFR in the MCF-7 cell after ARF6 depletion is not due to a defect in exosomal secretion. Plasma membrane levels of EGFR were not reduced in ARF6-depleted cells, as shown by biotinylation experiments ( Fig. 4d and Supplementary Fig. 4b,c ). The main difference was a higher content of intracellular EGFR in ARF6-depleted cells ( Fig. 4d ; Supplementary Fig. 4b,c ). Finally, ARF6-depleted cells were not less efficient in internalizing EGFR upon EGF stimulation ( Fig. 4d ; Supplementary Fig. 4b,c ). Taken together, these data indicate that ARF6 depletion impairs the post-internalization degradation of EGFR and suggests that ARF6 might also function in late endosomal trafficking of EGFR towards lysosomes. 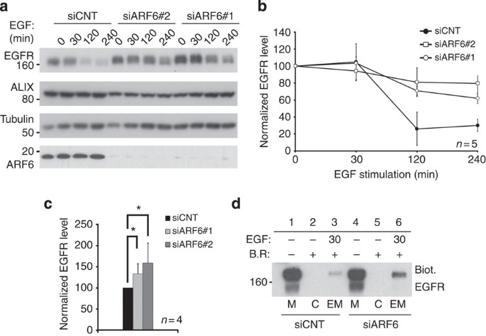Figure 4: ARF6 depletion reduces EGFR degradation. (a) Control or ARF6-depleted MCF-7 cells were starved for 3 h and treated with EGF (100 ng ml−1) as indicated. Cell lysates were analysed by western blotting. (b) Effect of EGF stimulation on the cellular levels of EGFR. EGFR levels were normalized with respect to tubulin or ALIX and to the signal at time 0. Values correspond to the relative mean intensities±s.d. (c) Histogram comparing the level of EGFR at steady state (time 0, no EGF stimulation) as measured by densitometry. Values correspond to the relative mean intensities±s.d. *P<0.05 (Student’st-test);n, number of independent experiments. (d) EGFR endocytosis from the plasma membrane upon EGF stimulation. Cells were biotinylated for 20 min. After 30 min (30) of EGF stimulation or not (−), biotin was reduced (+) or not (−). Biotinylated proteins from total cell extracts were captured with an avidin resin before EGFR detection by western blotting. Biotin reduction was totally effective (lane 1 versus 2 and 4 versus 5). Internalization of biotinylated EGFR is not reduced upon ARF6 depletion (lanes 6 and 3); see alsoSupplementary Fig. 4b,c. M, EGFR at the plasma membrane, C, control of biotin reduction, EM, EGFR endocytosed from the plasma membrane, B.R, biotin reduction, Biot. EGFR, biotinylated EGFR. Figure 4: ARF6 depletion reduces EGFR degradation. ( a ) Control or ARF6-depleted MCF-7 cells were starved for 3 h and treated with EGF (100 ng ml −1 ) as indicated. Cell lysates were analysed by western blotting. ( b ) Effect of EGF stimulation on the cellular levels of EGFR. EGFR levels were normalized with respect to tubulin or ALIX and to the signal at time 0. Values correspond to the relative mean intensities±s.d. ( c ) Histogram comparing the level of EGFR at steady state (time 0, no EGF stimulation) as measured by densitometry. Values correspond to the relative mean intensities±s.d. * P <0.05 (Student’s t -test); n , number of independent experiments. ( d ) EGFR endocytosis from the plasma membrane upon EGF stimulation. Cells were biotinylated for 20 min. After 30 min (30) of EGF stimulation or not (−), biotin was reduced (+) or not (−). Biotinylated proteins from total cell extracts were captured with an avidin resin before EGFR detection by western blotting. Biotin reduction was totally effective (lane 1 versus 2 and 4 versus 5). Internalization of biotinylated EGFR is not reduced upon ARF6 depletion (lanes 6 and 3); see also Supplementary Fig. 4b,c . M, EGFR at the plasma membrane, C, control of biotin reduction, EM, EGFR endocytosed from the plasma membrane, B.R, biotin reduction, Biot. EGFR, biotinylated EGFR. Full size image ARF6 is not involved in ESCRT-dependent HIV-1 budding Defects in ILV formation observed in ARF6-depleted cells might be suggestive of defective ESCRT machinery. To test this possibility, we investigated whether ARF6 depletion affects viral budding. Indeed, budding of retroviruses relies on ESCRTs to be effective at the plasma membrane and/or in MVBs [30] . During HIV-1 assembly, Gag molecules recruit components involved in various steps of the ESCRT pathway (that is, TSG101, NEDD4L, ALIX). This recruitment ultimately mediates a membrane fission step required for virion release [31] . In the absence of those components, Gag remains connected to the plasma membrane and the budding does not occur [32] . It was reported that ARF6 depletion does not affect cell infection by HIV-1 vectors pseudotyped with the VSV-G protein [33] . To determine whether ESCRT machinery involved in viral budding was functionally affected or not by ARF6 depletion, we infected MCF-7 cells, depleted or not for ARF6, with VSV-pseudotyped replication competent HIV-1. ARF6 depletion was verified to be and remain effective for the 6-day time course of the experiment ( Fig. 5a ). To study viral budding, the production of mature viral particles by infected MCF-7 cells was tested by immunofluorescence [34] . Non-permeabilized fixed cells were stained for cell surface Env. Cells were then permeabilized and stained with anti-MAp17 ( Fig. 5b ). This antibody detects only the cleaved matrix protein MAp17 and therefore labels mature virus particles. MAp17 signals were found at the plasma membrane and were barely detectable inside the cell, indicating that viral budding mainly occurs at the plasma membrane. The colocalization between Env and MAp17 confirmed that the viral material accumulated at cell periphery corresponds to mature viruses present at the cell surface. We quantified the amount of mature virus released from the cell surface by measuring the total fluorescence of MAp17 staining per cell nucleus ( Fig. 5c ) and observed no significant difference between control and ARF6-depleted cells. Consistently, cellular viral content ( Fig. 5d ) and viral release in the supernatant ( Fig. 5e ) were also similar. These results indicate that ARF6 depletion does not result in a general failure of ESCRT. 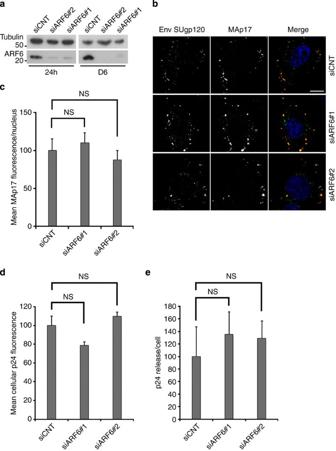Figure 5: ARF6 depletion does not affect viral budding. (a) Western blot illustrating sustained ARF6 depletion during the time course of the experiment, viral release being measured 6 days after RNAi treatment. (b,c) MCF-7 cells infected with VSV-G-pseudotyped HIV-1 were analysed by confocal fluorescence microscopy to test for their ability to allow viral budding. (b) Viral envelope proteins were stained with anti-Env SUgp120 antibodies (green) and viruses that completed their budding were detected with an antibody recognizing mature matrix protein MAp17 (red). Note the high level of colocalization illustrating that most virions completed their budding at the plasma membrane. Scale bar, 5 μm. Nuclei were stained with DAPI (blue). (c) The total MAp17 fluorescence was divided by the total number of nuclei in each field, calculated for 150 to 200 cells in three independent experiments. Histograms represent the mean fluorescence intensity per nucleus±s.d. as an estimation of the number of mature viruses released per cell. NS, non significant (Student’st-test). (d) After RNAi treatment, MCF-7 cells were infected with VSV-G-pseudotyped HIV-1. Three days after infection, cells were analysed by confocal fluorescence microscopy using a p24 antibody to stain intracellular Gag and the mature virus. The total p24 fluorescence was divided by the total number of nuclei in each field, calculated for 150 to 200 cells in three independent experiments. Histograms represent the mean fluorescence intensity per nucleus±s.d. NS, non significant (Student’st-test). (e) Virus release was determined by CAp24 quantification in the supernatant, using a HIV-1 p24 ELISA kit. p24 release was divided by the total number of cell. Results were normalized to 100% in siCNT cells. NS, non significant (Student’st-test). Figure 5: ARF6 depletion does not affect viral budding. ( a ) Western blot illustrating sustained ARF6 depletion during the time course of the experiment, viral release being measured 6 days after RNAi treatment. ( b , c ) MCF-7 cells infected with VSV-G-pseudotyped HIV-1 were analysed by confocal fluorescence microscopy to test for their ability to allow viral budding. ( b ) Viral envelope proteins were stained with anti-Env SUgp120 antibodies (green) and viruses that completed their budding were detected with an antibody recognizing mature matrix protein MAp17 (red). Note the high level of colocalization illustrating that most virions completed their budding at the plasma membrane. Scale bar, 5 μm. Nuclei were stained with DAPI (blue). ( c ) The total MAp17 fluorescence was divided by the total number of nuclei in each field, calculated for 150 to 200 cells in three independent experiments. Histograms represent the mean fluorescence intensity per nucleus±s.d. as an estimation of the number of mature viruses released per cell. NS, non significant (Student’s t -test). ( d ) After RNAi treatment, MCF-7 cells were infected with VSV-G-pseudotyped HIV-1. Three days after infection, cells were analysed by confocal fluorescence microscopy using a p24 antibody to stain intracellular Gag and the mature virus. The total p24 fluorescence was divided by the total number of nuclei in each field, calculated for 150 to 200 cells in three independent experiments. Histograms represent the mean fluorescence intensity per nucleus±s.d. NS, non significant (Student’s t -test). ( e ) Virus release was determined by CAp24 quantification in the supernatant, using a HIV-1 p24 ELISA kit. p24 release was divided by the total number of cell. Results were normalized to 100% in siCNT cells. NS, non significant (Student’s t -test). Full size image PLD2 is specifically implicated in ARF6 exosome biogenesis We then aimed to identify ARF6 effectors involved in ILV budding. We used the Ce-RAB5(Q79L) assay and efficient silencing ( Supplementary Fig. 5a,b ) as a rapid read-out of ILV formation inside endosomes to monitor the impact of different ARF6 effectors, in particular the PIP5Ks and PLDs [35] , [36] . Confocal microscopy revealed that mCh-syntenin filled the lumen of Ce-RAB5(Q79L) endosomes in MCF-7 cells depleted for PIP5Ks or PLD1 (86% for PIP5Kα, 94% for PIP5Kγ and 93% for PLD1; Fig. 6a,b and d ), suggesting that these effectors are not controlling ILV budding in the ARF6-syntenin-exosomal pathway. In contrast, PLD2 depletion drastically reduced mCh-syntenin enrichment inside Ce-RAB5(Q79L) endosomes, with only 29% mCh-syntenin filled endosomes left ( Fig. 6b,d ). Consistently, cells transiently co-transfected with Ce-RAB5(Q79L) and HA-PLD2 show that PLD2 is found at the limiting membrane of RAB5(Q79L) endosomes ( Supplementary Fig. 5c ). Similar to ARF6, this suggests a role for PLD2 at the limiting membrane of MVBs. The specific effect of PLD2 on mCh-syntenin endosomal budding was confirmed by using isoform selective PLD inhibitors. Indeed, confocal microscopy revealed that 85% of RAB5(Q79L) endosomes were filled with mCh-syntenin in MCF-7 cells treated with a PLD1 inhibitor ( Fig. 6c,d ), whereas this level was reduced to 49% in cells treated with a PLD2 inhibitor ( Fig. 6c,d ). Moreover, we analysed the exosomal release of cells treated with a PLD2 specific inhibitor by western blot ( Fig. 6e,f ). The amount of exosomal syntenin, ALIX and CD63 was significantly decreased (by 39%, 18%, and 44%, respectively). Notably, more than one-third of the total PLD activity was inhibited in ARF6-depleted cells ( Supplementary Fig. 5d ), indicating that in MCF-7 cells PLD activity is significantly under the control of ARF6. PLD2 metabolizes phosphatidylcholine (PC) into phosphatidic acid (PA) and choline. Strikingly, the PA-binding domain of Spo-20 (PABD-Spo20), a biosensor that specifically binds to PA [37] , decorates the limiting membrane of Ce-RAB5(Q79L) endosomes, suggesting that PA synthesis may occur at this location ( Supplementary Fig. 6a ). PLD2-depleted cells were analysed for their lipid content by HPLC-MS/MS, and a significant decrease in cellular PA was found ( Supplementary Fig. 6b ). Low amounts of PA could also be detected in exosomes; however, no significant difference in exosomal PA was detected upon PLD2 depletion ( Supplementary Fig. 6c ). Interestingly, syntenin and in particular its PDZ1 domain can directly interact with PA ( Supplementary Fig. 6d ). Altogether, these data suggest that PLD2 is the effector of ARF6 involved in ILV formation. 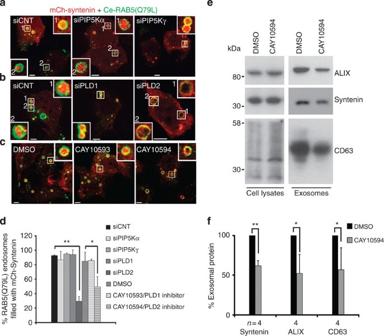Figure 6: Identification of ARF6 effectors implicated in syntenin intraendosomal budding. Confocal micrographs of MCF-7 cells treated with non-targeting RNAi (siCNT), or with RNAi targeting PIP5Kα, PIP5Kγ, PLD1 or PLD2 (a,b). Cells were transiently transfected with expression vectors for Ce-RAB5(Q79L) (green) and mCh-syntenin (red) 48 h after RNAi treatment and analysed 24 h later. Note the concentration of mCh-syntenin inside the lumen of the enlarged endosomes outlined by Ce-RAB5(Q79L) (see insets for higher magnification of individual endosomes) in all cells except in PLD2-depleted cells. (c) Confocal micrographs of MCF-7 cells treated with DMSO as control, the PLD1 inhibitor CAY10593 (10 μM) or the PLD2 inhibitor CAY10594 (10 μM). Cells were transiently transfected with expression vectors for Ce-RAB5(Q79L) (green) and mCh-syntenin (red) for 24 h in the presence of drugs or solely DMSO. Note the absence of mCh-syntenin inside the Ce-RAB5(Q79L) endosomes, solely in cells treated with the drug inhibiting PLD2. (d) Quantification of the number of Ce-RAB5(Q79L) endosomes filled with mCh-syntenin±s.d. Three independent experiments were performed and at least 30 RAB5(Q79L) endosomes were examined in each experiment. Scale bars, 5 μm. (e) MCF-7 cells were treated with DMSO as control or the PLD2 inhibitor CAY10594 (10 μM). Total cell lysates and the corresponding exosomes were analysed by western blotting for different markers, as indicated. Note the reduction of exosomal markers upon PLD2 inhibition (f) Histograms represent mean signal intensities±s.d. in exosomes produced by cells treated with CAY10594, relative to signals in exosomes produced by cells treated with DMSO, calculated for four independent experiments. *P<0.05, **P<0.01 (Student’st-test). Figure 6: Identification of ARF6 effectors implicated in syntenin intraendosomal budding. Confocal micrographs of MCF-7 cells treated with non-targeting RNAi (siCNT), or with RNAi targeting PIP5Kα, PIP5Kγ, PLD1 or PLD2 ( a , b ). Cells were transiently transfected with expression vectors for Ce-RAB5(Q79L) (green) and mCh-syntenin (red) 48 h after RNAi treatment and analysed 24 h later. Note the concentration of mCh-syntenin inside the lumen of the enlarged endosomes outlined by Ce-RAB5(Q79L) (see insets for higher magnification of individual endosomes) in all cells except in PLD2-depleted cells. ( c ) Confocal micrographs of MCF-7 cells treated with DMSO as control, the PLD1 inhibitor CAY10593 (10 μM) or the PLD2 inhibitor CAY10594 (10 μM). Cells were transiently transfected with expression vectors for Ce-RAB5(Q79L) (green) and mCh-syntenin (red) for 24 h in the presence of drugs or solely DMSO. Note the absence of mCh-syntenin inside the Ce-RAB5(Q79L) endosomes, solely in cells treated with the drug inhibiting PLD2. ( d ) Quantification of the number of Ce-RAB5(Q79L) endosomes filled with mCh-syntenin±s.d. Three independent experiments were performed and at least 30 RAB5(Q79L) endosomes were examined in each experiment. Scale bars, 5 μm. ( e ) MCF-7 cells were treated with DMSO as control or the PLD2 inhibitor CAY10594 (10 μM). Total cell lysates and the corresponding exosomes were analysed by western blotting for different markers, as indicated. Note the reduction of exosomal markers upon PLD2 inhibition ( f ) Histograms represent mean signal intensities±s.d. in exosomes produced by cells treated with CAY10594, relative to signals in exosomes produced by cells treated with DMSO, calculated for four independent experiments. * P <0.05, ** P <0.01 (Student’s t -test). Full size image To evaluate the specific role of PLD2 in exosomal release, we analysed the exosomes secreted by PLD1- and PLD2-depleted cells ( Fig. 7a,b ). Two different RNAis targeting PLD2 decreased the amount of syntenin, ALIX and CD63 in exosomes (by 52%, 63% and 77%, respectively). In contrast, no significant difference in the exosomal release of these markers was observed for PLD1 silencing. The ultrastructure of MVBs in PLD1- and PLD2-depleted cells was further investigated by electron microscopy. As observed in syntenin and ARF6-depleted cells, CD63-HRP staining was found to be associated with limiting membranes and on ILVs that were peripherally located, but the lumen of the endosomes remained largely empty ( Fig. 7c,d ). Of note, PLD1-depleted cells presented no significant defect in CD63-HRP staining compared with CNT cells ( Fig. 7c , middle panel), indicating that the ILVs are correctly formed in these cells. Taken together, these results show that PLD2 is specifically required for ILV formation and syntenin exosome biogenesis. 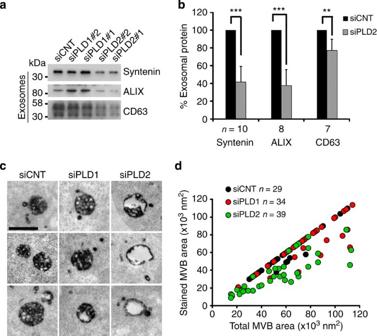Figure 7: PLD2 but not PLD1 controls syntenin exosomal release and CD63 ILV budding. (a) MCF-7 cells were treated with two different PLD1 or PLD2 RNAi (siPLD1#1, siPLD1#2, siPLD2#1 and siPLD2#2) or non-targeting RNAi (siCNT). PLD1 or PLD2 depletion did not affect cell growth within the first 48 h. Exosomes were analysed by western blot using different markers as indicated. (b) The histogram represents mean signal intensities±s.d. in exosomes, relative to signals in siCNT exosomes, calculated fornindependent experiments in cells depleted for PLD2. siPLD2#1 and siPLD2#2 data were pooled for quantification and statistical analysis. **P<0.01, ***P<0.001 (Student’st-test). (c) Representative electron micrographs, illustrating the morphology of the late endosomal compartment in MCF-7 cells treated with a pool of four RNAi for PLD1 (siPLD1) or PLD2 (siPLD2) or non-targeting RNAi (siCNT), as indicated. Structures were revealed by peroxidase-conjugated anti-CD63 internalization for 30 min, and staining with DAB. Scale bar, 500 nm. (d) Endosome filling; quantification as inFig. 3;nis the total number of endosomes examined in three independent experiments. Figure 7: PLD2 but not PLD1 controls syntenin exosomal release and CD63 ILV budding. ( a ) MCF-7 cells were treated with two different PLD1 or PLD2 RNAi (siPLD1#1, siPLD1#2, siPLD2#1 and siPLD2#2) or non-targeting RNAi (siCNT). PLD1 or PLD2 depletion did not affect cell growth within the first 48 h. Exosomes were analysed by western blot using different markers as indicated. ( b ) The histogram represents mean signal intensities±s.d. in exosomes, relative to signals in siCNT exosomes, calculated for n independent experiments in cells depleted for PLD2. siPLD2#1 and siPLD2#2 data were pooled for quantification and statistical analysis. ** P <0.01, *** P <0.001 (Student’s t -test). ( c ) Representative electron micrographs, illustrating the morphology of the late endosomal compartment in MCF-7 cells treated with a pool of four RNAi for PLD1 (siPLD1) or PLD2 (siPLD2) or non-targeting RNAi (siCNT), as indicated. Structures were revealed by peroxidase-conjugated anti-CD63 internalization for 30 min, and staining with DAB. Scale bar, 500 nm. ( d ) Endosome filling; quantification as in Fig. 3 ; n is the total number of endosomes examined in three independent experiments. Full size image In this study, we identify ARF6 as a regulator of the production of syntenin exosomes. We show that ARF6 inhibition in cells leads to a significant decrease in exosomal proteins. Moreover, the fast cycling mutant ARF6-T157N increases and rescues syntenin exosomal secretion, indicating that the GDP/GTP complete cycle of ARF6 is crucial for stimulating exosome production. Among the ARF6 GEFs, we obtained evidence that ARNO might be more directly implicated in the control of ARF6-dependent exosomal secretion. ARF6 has been implicated in the endocytosis of several membrane proteins [29] , [38] . Here we show that ARF6 depletion does not influence the internalization rate of the syntenin cargo CD63. Rather, CD63 accumulates in intracellular compartments. CD63 does not accumulate in early endosomes, which indicates that the effect of ARF6 on exosome production cannot be explained by a defect in early endocytosis. CD63 does not accumulate in recycling endosomes either. Electron microscopy provided no evidence for impaired fusion of MVB with the plasma membrane as we did not observe CD63-MVB accumulation near the plasma membrane. This differentiates ARF6 from the small GTPases RAB27 and RAB35, which were previously shown to control exosome secretion at this step [39] , [40] . In ARF6-depleted cells, CD63 concentrates at the level of LAMP2 late endosomes. Electron microscopy experiments allowed to show that ARF6 is necessary for CD63 intraluminal budding into MVBs. Loss of ARF6 does not affect the size, but the filling of the endosome stained with CD63. A difficulty for cells to produce and secrete exosomal CD63 upon ARF6 downregulation would explain CD63 accumulation in the cells and in particular in late endosomal compartments presenting a defect in ILV formation. Taken together, the data indicate that ARF6 is not implicated in the delivery of cargo to late endosomes but in the formation of ILVs. Intriguingly, ARF6 depletion does not seem to block all ESCRT-dependent processes as HIV budding is not affected. Yet, we cannot exclude that ARF6-dependent intraluminal budding is ESCRT-dependent, as the syntenin exosomal pathway depends on ALIX and some ESCRT components [16] . In this context, it has been shown that EGF treatment specifically upregulates ESCRT-dependent ILV formation [41] . Here we show that ARF6 controls EGFR late endosomal sorting as its depletion results in increased cellular EGFR and in a lack of EGFR degradation upon EGF stimulation. In ARF6-depleted cells, EGFR accumulates inside the cell. Recycling defects can apparently be excluded as ARF6 depletion does not reduce plasma membrane EGFR. Thus, ARF6 also seems to have an impact on the formation of degradative late endosomes (destined for fusion with lysosomes, with ILV degradation) and by extension on related ESCRTs. Interestingly, it has recently been shown that the ARF6 effector PIP5K (specifically the gamma i5 isoform) is required for the EGFR sorting into ILVs of the MVB upon EGF stimulation in MDA-MB-231 cells [42] . This was dependent on the ESCRT component Hrs. Yet it was not investigated whether this was dependent on ARF6 and whether this PIP5K might affect exosomal release. Depletion of PIP5K gamma did not have an impact on syntenin endosomal budding, but levels of this enzyme are low in MCF-7 cells. Indeed, looking for ARF6 effectors that might support syntenin exosomal production, we tested the various PIP5Ks and PLDs isoforms expressed in MCF-7 cells for their effect on endosomal budding. We found no evidence for a role of any of the PIP5Ks in syntenin endosomal budding. This is somehow consistent with a general role for ARF6-PIP5K in endosomal recycling from the perinuclear compartment to cell surface [43] and in particular with a role for ARF6-PIP5K in the plasma membrane recycling of the syntenin-PDZ cargo syndecan in a syntenin-phosphatidylinositol 4,5-phosphate (PI(4,5)P2)-dependent manner [26] . Two isoforms of mammalian PLD, PLD1 and PLD2 have been identified [44] . Although PLD1 was previously shown to be localized to late endosomes and lysosomes [45] , our observations exclude a role for PLD1 in the ARF6-syntenin exosomal pathway. On the contrary, we established a clear role for PLD2 in ILV budding and syntenin exosomes. In some circumstances, ARF6 has been shown to selectively stimulate PLD2 activity [46] , but to our knowledge no role for PLD2 in late endosomal trafficking has been documented; nevertheless, PLD2 was reported to be enriched and specifically sorted on exosomes when overexpressed in RBL-2H3 cells [47] . Interestingly, ARF6 has been implicated in the shedding of microvesicles from the plasma membrane, and the data also suggest a role for PLD in this process [48] . Yet, this was done with different methodological approaches and in different cells. It might thus be that, depending on the signalling context, ARF6-PLD exerts the same topological effects (budding from the cytosol) at different subcellular locations, such as the plasma membrane or the endosomal membrane. PLDs are known to metabolize phosphatidylcholine into phosphatidic acid (PA). With a very small negatively charged headgroup close to the acyl chains, PA generated in the inner leaflet of membranes is likely to induce a negative membrane curvature [49] , which might favour endosomal intraluminal budding. In the same manner, the cone-shaped structure of ceramide may induce spontaneous negative curvature in the membrane bilayer promoting membrane invagination [14] . Local lipid compositions that might reorganize into specialized endosomal regions might induce membrane bending and induce ILV formation. Indeed, it has been shown that lipids and a pH gradient are sufficient to form ILVs in LBPA-containing liposomes [50] . We found that a PA probe enriches at the limiting membrane of RAB5(Q79L) endosomes that can undergo endosomal budding and create giant ‘MVB-like’ organelles [28] . Moreover, syntenin can directly interact with PA, which might support syntenin-ALIX complexes to be sorted in PA-enriched lipid microdomains. It is thus tempting to speculate that the product of PLD2 activity, PA, is directly involved in ILV budding. PLD2-depleted cells were analysed by HPLC-MS/MS for their lipid content and present a significant decrease in total cellular PA level. We also found that exosomes contain low levels of PA that were not affected by PLD2 silencing. This might be because the PLD2-generated PA required for exosome production might be restricted to nascent budding ILVs, consistent with the localization of the PA probe at the limiting membrane but not inside RAB5(Q79L) endosomes. It is also worth to mention that PA can be produced through various biosynthetic pathways that include PLD1/2, up to 10 diacylglycerol kinases and various lysophosphatidic acid acyl-transferases. Therefore, the exact source of the PA detected on exosomes remains to be directly established. Altogether an appealing model would be that ARF6-PLD2-PA controls syntenin-ALIX ILV formation and thereby subsequent exosomal release, with effects on ESCRTs that are selective or depend on context (that is, specific cargo). Expression vectors and reagents For gain-of-function studies in cells, the cDNA encoding full-length non-tagged syntenin was cloned in pcDNA3.1/Zeo(+) (Invitrogen). The cDNA encoding mCherry-syntenin was derived from the eGFP-syntenin cDNA construct [19] , by restriction ligation. The expression vector for Ce-RAB5(Q79L) was received from W. Annaert (K.U. Leuven, Belgium) and non-tagged ARF6-WT and ARF6-T157N constructs were generated from mCherry-tagged forms provided by M. Franco (IPMC, Sophia Antipolis). For the rescue experiments, we used open-reading frames where we generated three point mutations in the target sequence of the siRNA. All constructs were verified by sequencing. All RNAi targeting human sequences (siGENOME and On-target plus) and the non-targeting control RNAi (siCNT) were purchased from Dharmacon Inc. ARF6#2 (5′-GGUCUCAUCUUCGUAGUGG-3′); ARF6#1 (5′-GCACCGCAUUAUCAAUGACCG-3′); PIP5K α RNAi (ON-TARGET plus Smart pool L-004780), syntenin (5′-GCAAGACCUUCCAGUAUAA-3′), PLD1 siGENOME SMARTpool (M-009413), PLD1#2 (5′-GAAGAACAAUUCCUUGGUA-3′), PLD1#1 (5′-GAAGAUUACUUGACAAAGA-3′), PLD2 siGENOME SMARTpool (M-005064), PLD2#2 (5′-GGACCGGCCUUUCGAAGAU-3′); PLD2#1 (5′-CAGCAUGGCGGGACUAUAU-3′). PIP5K γ RNAis (PAN targeting specifically isoform 1 and 2 and RNAis targeting isoform 5) were kindly provided by R. Anderson (Madison, USA). qPCR primer sequences are supplied in Supplementary Table 1 . Anti-syntenin, anti-syndecan-1CTF and anti-ALIX antibodies were as described earlier [16] . Other antibodies were from commercial sources and were used as recommended by the manufacturers. Antibodies directed against CD63 (MEM-259) was from Abcam (dilution 1/500), Tubulin (T6199) from Sigma-Aldrich (dilution 1/10,000), EEA1 (610456) from BD Biosciences (dilution 1/250), LAMP2 (PA1-655) from Thermo Scientific (dilution 1/2,000), EGFR from Cell Signaling (2,232, dilution 1/1,000), SUgp120 from NIH AIDS Research (clone 2G12, used at 0,5 μg ml −1 ), HIV-1SF2 p24 Antiserum from NIH AIDS Research (catalogue number 4250, dilution 1/500), MAp17 from Hybridolab (clone 18A, dilution 1/500) and ARF6 was from Santa Cruz (sc-7971, dilution 1/500). The CAY10593 inhibitor (used at 10 μM) was purchased from Cayman Chemical (13206) and the CAY10594 inhibitor (used at 10 μM) from Santa Cruz (sc-223874). Statistical analysis was performed using the standard two-tailed Student t -test, and * P <0.05, ** P <0.01, *** P <0.001 were considered statistically significant. Cells and transfections MCF-7 cells were obtained from ATCC (Manassas, VA). Cells were routinely grown in DMEM/F12 (1:1) medium (Life technologies, Gaithersburg, MD) supplemented with 10% fetal calf serum (FCS) (Hyclone, Logan, UT). Serum used for experiments was depleted of exosomes, by prior overnight centrifugation at 140,000 × g . For transient expressions, the cells were transfected the day after plating using Fugene HD reagent (Roche). For RNAi experiments, cells at a confluence of 50% were transfected with 20 nM RNAi using Lipofectamine RNAiMAX reagent (Life technologies, USA); cells were analysed 48 or 72 h after RNAi treatment. For drug treatment, cells were simultaneously treated with the PLD1 inhibitor CAY10593 or the PLD2 inhibitor CAY10594 and transiently transfected to coexpress mCh-syntenin with Ce-RAB5(Q79L), for 24 h. Exosomes and total cell lysates For comparative analyses, in gain- and loss-of-function studies, exosomes were collected from equivalent amounts of culture medium, conditioned by equivalent amounts of cells. After the required time of cDNA or RNAi treatments, the cell layers were washed twice with PBS and refreshed with DMEM/F12 containing 10% exosome-depleted FCS. Cell-conditioned media were collected 16 h later. Exosomes were isolated from these media by three sequential centrifugation steps at 4 °C: 10 min at 500 × g , to remove cells; 30 min at 10,000 × g , to remove cell debris; and 3 h at 140,000 × g , to pellet exosomes, followed by one wash (suspension in PBS/centrifugation at 140,000 × g ), to remove soluble serum and secreted proteins. Exosomal pellets prepared by differential HSC exosomes were then re-suspended in lysis buffer (PBS supplemented with 1% NP40, 10 mM EDTA and protease inhibitor cocktail containing 1 μg ml −1 antipain, 1 μg ml −1 pepstatin, 15 μg ml −1 benzamidine and 1 μg ml −1 leupeptin). The corresponding cell layers were washed in cold PBS and scraped on ice. Lysates from corresponding cultures were cleared by centrifugation at 300 × g for 5 min at 4 °C and then re-suspended in lysis buffer. Although little variations were observed from sample to sample (max 10%), exosomal amount loaded for the western blot was normalized according to the number of parent cells from where exosomes were secreted. EGFR internalization MCF-7 cells were transfected with either siCNT or siARF6#2. After 48 h of transfection, cells were washed three times with PBS+MgCl 2 and biotinylated for 20 min with reducible sulfo-NHS-SS-biotin (Pierce) at 4 °C. After stimulation with EGF 100 ng ml −1 , cell surface biotin was removed by treatment (2 × 20 min) at 4 °C with sodium 2-mercaptoethanesulphonate (MesNa, Sigma). To determine the intracellular pools of biotinylated receptors, cells were lysed and incubated with avidin resin (Thermo Scientific). After capture and washes, the complexes were separated by SDS–PAGE and EGFR was detected by western blot. Signals were detected by chemiluminescence and quantified using ImageJ (National Institutes of Health, Bethesda, MD, USA). Western blotting The proteins were heat-denaturated in Laemmli sample buffer and fractionated in 12.5% gels by SDS–PAGE, electro-transferred to nitrocellulose membrane, stained with Ponceau red and immunoblotted with the indicated antibodies. Signals were visualized with enhanced chemiluminescence detection reagent (Amersham Pharmacia Biotech) and were quantified by densitometric scanning, using ImageJ. Full scans of all western blots are supplied in Supplementary Fig. 7 . CD63 internalization MCF-7 cells were treated with siCNT or siARF6 and plated in 24-well dishes at a concentration of 100,000 cells per well. After 72 h, the cells were incubated for 30 min at 4 °C with 2 μg ml −1 anti-CD63 antibody in complete media, washed twice in PBS and then incubated at 37 °C. At each time point, cells were washed with PBS and fixed with 4% paraformaldehyde (PFA), 15 min at RT and incubated 30 min in PBS containing 3% BSA and 0.05% saponin with Alexa-488 donkey anti-mouse IgG and Hoechst. The anti-CD63 internalized was estimated by confocal microscopy, using one focal plane. The percentage of internal CD63 was measured by ImageJ. Immunofluorescence staining and confocal microscopy Cultured cells on glass coverslips were fixed with 4% PFA for 15 min, washed in PBS and then incubated with the indicated antibodies with PBS containing 3% BSA and 0.05% saponin. Coverslips were mounted on DABCO/Mowiol and observed with a Zeiss Meta confocal microscope (LSM 510 META, Zeiss, France) with a UV laser and × 63 objectives. Confocal images were analysed using ImageJ and Photoshop (Adobe, San Jose, CA) software. Electron microscopy For the MVB morphology studies, cells were incubated for 30 min at 37 °C with an anti-CD63 antibody (Abcam) labelled with horseradish peroxidase (Z 25054 Molecular Probes). The cells were then washed with PBS and fixed for 1 h in 3% glutaraldehyde in 0.1 M sodium cacodylate (NaCaC) buffer. After several washes in 0.1 M NaCaC, the cells were incubated with diaminobenzidine (DAB; Sigma) in 0.05 M Tris-HCl, pH 7.6. The enzymatic reaction was initiated by adding H 2 O 2 at a final concentration of 0.01% and allowed to proceed for 30 min. After washing in Tris-HCl buffer, the cells were post-fixed for 1 h with 1% osmium tetroxide in 0.1 M phosphate buffer, washed, scraped, re-suspended in 2% agar and pelleted. Sliced agar blocks were dehydrated in a series of ethanol and embedded in Agar 100 resin polymerized for 48 h at 60 °C. sixty nanometre sections (Ultracut E Leica) were counterstained with 2% uranyl acetate and lead citrate (Reynold’s), and were examined with a ZEISS EM 912 and images were taken with a gatan Bioscan camera. MVBs sectional areas were measured using ImageJ software, and the data were analysed using Excel software. HIV-1 assays Wild-type replication competent viruses (HIV NL4.3 WT), pseudotyped with vesicular stomatitis virus envelope glycoprotein (VSV-G) were produced in HEK293T cells by transient transfection with a 5:1 plasmid ratio, using the calcium-phosphate precipitation technique. Three days after transfection, viruses were collected, frozen and kept for further application. Virus concentration was determined by CAp24 quantification in the supernatant, using a HIV-1 p24 ELISA kit (PerkinElmer Life Science, Inc.). MCF-7 cells were transfected with either siCNT, siARF6#1 or siARF6#2 as described above and grown in 24-well plates, on coverslips. After 3 days, 2 × 10 5 MCF-7 cells were infected with 50 ng of Cap24-pseudotyped virus. Cells were washed four times, 4 h after infection. Three days after infection, infected cells on coverslips were washed and fixed with 4% PFA in PBS for 20 min. For extracellular staining of Env, cells were incubated for 1 h at RT with anti-Env HIV-1 gp120 IgG1κ mouse monoclonal antibody (clone 2G12, NIH AIDS Research and Reference Reagent Programme, Division of AIDS, NIAID). Mature viral particles were stained using an anti-MAp17 IgG2a mouse monoclonal antibody (clone 18A, Hybridolab) in PBS containing 1% BSA and 0.1% triton-X100. Cells were then washed and labelled with a FITC-conjugated goat anti-mouse-IgG1 antibody (SouthernBiotech) and Cy3-conjugated goat anti-mouse-IgG2a (Jackson Immunoresearch), followed by Alexa488-conjugated goat anti-FITC (Molecular Probes). After wash in PBS, coverslips were mounted in ProLong Gold antifade reagent with DAPI (Life Technologies). Confocal images were obtained using a LSM 700 confocal microscope (Carl Zeiss) over a × 63 objective. Z-stack optical sections were acquired at 0.2 μm depth increments for imaging or 1 μm increments for quantification. For quantification, cells were randomly chosen and about 10 contiguous optical sections contained the whole-cell fluorescence information. Both green and red laser excitation were intercalated to minimize cross-talk between the acquired fluorescence channels. Analysis of viral budding was performed using ImageJ. Viral release per cell was determined by CAp24 quantification in the supernatant, using a HIV-1 p24 ELISA kit (PerkinElmer Life Science, Inc.) divided by the number of cells. Lipid overlay assays GST and GST-tagged Syntenin-PDZ1 domain were produced in E. Coli (ER2566) and purified with glutathione beads. Overlay assays were performed as described in ref. 51 . 100 pmol lipids were immobilized on the nitrocellulose membrane. The fat-free milk blocked membranes were incubated with 5 μg ml −1 GST-tagged proteins. Bound proteins were detected using the primary anti GST antibody, HRP-conjugated secondary antibody and ECL detection. How to cite this article: Ghossoub, R. et al. Syntenin-ALIX exosome biogenesis and budding into multivesicular bodies are controlled by ARF6 and PLD2. Nat. Commun. 5:3477 doi: 10.1038/ncomms4477 (2014).